Magnetic monopoles and unusual dynamics of magnetoelectrics The modelling of magnetic monopoles in solids is a hot topic nowadays. Here, I propose that in solids with the linear magnetoelectric effect there should exist, close to electric charges, magnetic textures of magnetic monopole type. Their existence can lead to rather striking consequences, such as (magneto)electric Hall effect, magnetophotovoltaic effect and so on, which can be observed experimentally. In addition, in ordinary magnetoelectric materials not only magnetic monopoles can accompany the charge, but also more complicated local magnetic objects can be created, for example, local toroics, which can also lead to unusual effects in transport and other properties of such systems. The quest for magnetic monopoles became a hot topic in condensed matter physics lately, both theoretically and experimentally [1] , [2] , [3] , [4] , [5] . Especially exciting is the suggestion of the appearance of magnetic monopoles on image charges in topological insulators [6] . However, the experimental setup proposed for their observation in ref. 6 is rather elaborate. These situations, however, are not the only ones in which one can model magnetic monopoles in solids. As I show below, magnetic monopoles should exist in much simpler and well studied systems—in linear magnetoelectrics such as Cr 2 O 3 (ref. 7 ) or in some multiferroics [8] . The possibility of having the linear magnetoelectric effect (ME)—magnetization M induced by electric field E , M ~ E , or electric dipoles or polarization P induced by magnetic field B , was first discussed by Landau and Lifshitz [9] and by Dzyaloshinskii [7] . Many properties of ME materials have been clarified since then. However, not much attention has been devoted to the electrodynamic and transport properties of these systems—most probably because to observe clearly the ME effect one requires good insulators; and conductivity (leakage currents) is usually treated as a nuisance that must be get ridden of. I argue that due to the presence of magnetoelectric coupling, there may appear quite interesting and at first glance counterintuitive effects in ME systems, in particular, in their transport properties. These effects are connected with the apparent appearance in these systems of magnetic textures around every electric charge, having properties of magnetic monopoles—analogous to monopole spin textures in spin ice [1] , [2] , [3] , [4] , [5] . The presence of such monopoles, that is, the fact that each electron, besides possessing electric charge e , can also be characterized by magnetic charge g , can significantly influence the electrodynamic response of such media. Many resulting effects can also be explained without using the notion of monopoles, but this notion turns out to be very useful, and provides a natural way of explaining and predicting many surprising effects. Magnetic monopoles at electric charge in a magnetoelectric The linear ME is connected with the presence of the term α E · B in the free energy of the system, or, more generally, of the term α ij E i B j (where we assume summation over repeated indices). The ME tensor α ij can have both symmetric and antisymmetric components. In the simplest case, when α ij = αδ ij , we recover the ME coupling α E · B . It is easy to see that in this case, every charge placed in such media, such as an electron or charge impurity, would create a magnetic monopole, see Fig. 1 : the electric field E ( r )=( e / r 2 )( r / r ) would create a radial magnetic polarization M = α E —exactly as for a magnetic monopole with magnetic charge g = αe (magnetic ‘hedgehog’). Thus this object, with both electric and magnetic charge, would be what in elementary particle physics is called a dyon [10] , [11] . If an electron would move through such media, the magnetic monopole would move with it, which can lead to interesting consequences and would allow to observe such monopoles. The resulting equations describing the dynamics of corresponding objects will be the same as those for an electric charge, with the substitution (electric charge e ↔magnetic charge g ; electric field E ↔magnetic field H ) and the linearity of the corresponding equations leads to the well-known principle of superposition, valid also for the magnetic charges. 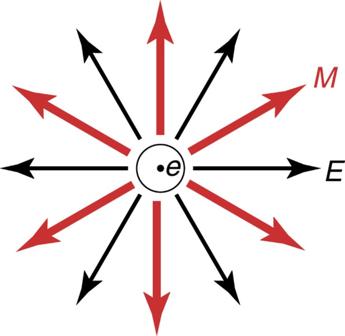Figure 1: Magnetic monopole created by a chargeein magnetoelectric media with the couplingαE·B. Black arrows denote force lines of the electric field, and red arrows show the resulting magnetization texture of the monopole type. Figure 1: Magnetic monopole created by a charge e in magnetoelectric media with the coupling α E · B . Black arrows denote force lines of the electric field, and red arrows show the resulting magnetization texture of the monopole type. Full size image Actually, the radial magnetic field around the charge is created by the corresponding deviations of ordered spins forming the ME material. Therefore, there will be no real singularity at the centre of the monopole. But the field outside the core will be exactly that of a magnetic monopole, and all the dynamic effects will be described by the usual dynamics with the electric charge e replaced by the magnetic charge g , and the electric field by H . There will also be no contradiction with the Maxwell equations: as in ref. 1 , the monopolar-like distribution of M , with non-zero divergence, will lead to a similar distribution of magnetic field H , so that the field B = H +4 π M will satisfy the standard Maxwell equation div B =0. A good classification of different electric and magnetic multipoles, in particular of their contribution to resonant X-ray scattering, is given by Lovesey and Scagnoli [12] . In particular, they noticed that the P -odd and T -odd scalar (actually pseudoscalar) multipole has all the properties of a magnetic charge, that is, a magnetic monopole. This points to a close relation between such monopoles and the ME phenomena, which also require broken both inversion symmetry and time-reversal invariance. However, the microscopic origin of the appearance of such monopoles in different situations, which is the main topic of the present paper, was not discussed in the otherwise very useful work [12] . Some dynamic consequences The presence of a magnetic charge of an electron could lead to many consequences. Thus, such monopole-like magnetic textures should exist around static charges in magnetoelectric media (charged impurities, defects, etc.) Mobile carriers, i.e., electrons, would start to move in a static magnetic field. If we put such a material with an extra electron in an external magnetic field H , there will indeed be a force F = g H acting on the monopole associated with the charge e , with magnetic charge g = αe , that is, the force will be F = αe H . In real situations, one can create mobile charge carriers in insulating magnetoelectrics by doping, by photoexcitation or by injection from the contacts; the temperature-induced electron and hole excitations would also manifest such properties. At small concentrations, one can always consider them independent. We can also explain the force acting on charges in magnetoelectrics in external magnetic field without invoking the notion of monopoles. Indeed, an external magnetic field creates in ME media an electric field E = α H , that is, the force will be F = g H =( αe ) H = e ( α H )= e E ; that is, it is the same force as that of an electric field acting on a charge. In this sense, the very motion of an electron in a magnetic field in a magnetoelectric is not a unique consequence of the appearance of magnetic monopoles. The question, however, is whether in this case both forces will act on the electron. Thus, if we apply an electric field to such a media, it will act on the electron by the force F = e E , but this external field will also create a magnetic field H = α E , and this magnetic field will also act on the magnetic monopole, with the force F′ = g H = eα 2 E . In effect, the effective force acting on the electron could be combined, F + F′ , or the electric charge of the electron could be renormalized, e → e (1+ α 2 ). One can also think of other interesting consequences. Thus, similar to the Lorentz force acting on a charge moving in a magnetic field, F ~ e [ υ × H ], which leads to the Hall effect, there will be a similar tangential force acting on a magnetic monopole moving in an electric field, F ~ g [ υ × E ]. Consequently, if we put a stripe of such ME material with a current in a perpendicular electric field, the monopole, together with the electron, would be deviated, exactly as in the Hall effect, see Fig. 2 . Such an ‘electric Hall effect’ should be observable in ME materials with diagonal ME coupling α ij = αδ ij and with magnetic monopoles. Once again, this may not be surprising: in such media, the electric field E perpendicular to the current will also create a magnetic field parallel to E , so that one can also attribute the Hall effect depicted in Fig. 2 to the ordinary Hall effect in this effective magnetic field H = α E . Still, this (magneto)electric Hall effect is an interesting special feature of such ME materials, which would be very interesting to study experimentally. 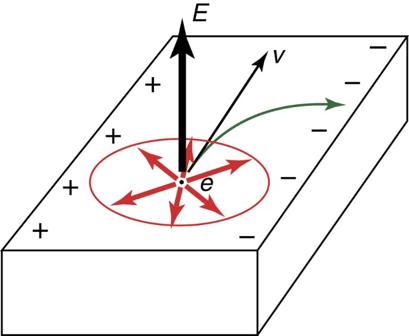Figure 2: Electric Hall effect. Motion of a magnetic monopoleg, accompanying the electric chargee, in a perpendicular electric field. The forceg[υ×E] will bend the trajectory of this object, leading to an ‘electric Hall effect’. Figure 2: Electric Hall effect. Motion of a magnetic monopole g , accompanying the electric charge e , in a perpendicular electric field. The force g [ υ × E ] will bend the trajectory of this object, leading to an ‘electric Hall effect’. Full size image One can think of some other effects connected with the dichotomy e ↔ g , E ↔ H . It was proposed in ref. 13 to use for topological insulators the analogy of the classical effect that the electric current creates a magnetic field around it: the motion of the magnetic monopole, if present, would similarly create an electric field around the ‘wire’ with the monopole current, which the authors of ref. 13 proposed to observe. The details of our situation are different: the corresponding magnetic field outside the topological insulator, looking like the field of a magnetic monopole, is actually created by dissipationless currents running on the surface of the topological insulator, whereas in our case it is created by a rearrangement of magnetic dipoles in the ME media. The resulting effect, however, would be similar. Yet another interesting effect may exist in such ME media under illumination. In ordinary ferroelectrics, there exists the well-known photovoltaic effect [14] : the electron–hole pairs created under illumination move in the internal electric field, existing in ferroelectrics, in opposite directions, thus creating a voltage. Similarly, in ME media with, for example, a diagonal ME tensor α ij = αδ ij , there should exist a similar effect caused by the magnetic field ( cf. Men'shenin and Turov [15] ): photoexcited electrons and holes would be accompanied by the corresponding monopoles with magnetic charges ± g , which would move in opposite direction in an external magnetic field, also leading to the voltage (magnetophotovoltaic effect). Magnetic textures close to charges in systems with toroidal moments The origin of the effects considered above conceptually is similar to that proposed for topological insulators [6] , although the resulting effects have here a bulk nature and seem to be more general and easier to observe. However, the ME media open yet other possibilities. The ME tensor α ij can have not only a symmetric, but also an antisymmetric part, which can be described by the dual vector—the toroidal, or anapole moment T . The resulting ME coupling can then be written as T ·[ E × B ]. Consequently, an electric charge placed in such media will create a local magnetic ‘toroic’—a magnetic vortex with the magnetic moment M ( r )~ T × E (with E =(4 πe / r 2 )( r / r )), see Fig. 3 . The moving electron will carry with itself such a ‘magnetic donut’. To detect it would be less easy than detecting magnetic monopoles: the toroidal moment couples not to H , but to curl H [16] , ~ T ·[ ∇ × H ]= T ·4 π j . Still, some interesting effects can be proposed. Thus, we can have in such media, for example, a spontaneous Hall effect like that shown in Fig. 2 , but even without a perpendicular external electric field: if the toroidal moment is perpendicular to the current j , such current would deviate so as to have a component parallel to T , decreasing the corresponding interaction energy. This would create a Hall voltage, see Fig. 4 . Again one can explain this simpler by saying that the applied voltage and the corresponding electric field E || j will create a magnetic field H ~ T × E , and in this magnetic field there will appear an ordinary Hall effect. Nevertheless, it is still a nontrivial effect, which would be interesting to study experimentally. There should be probably some other unusual effects connected with the presence of toroidal moments in the system, which are worth exploring. 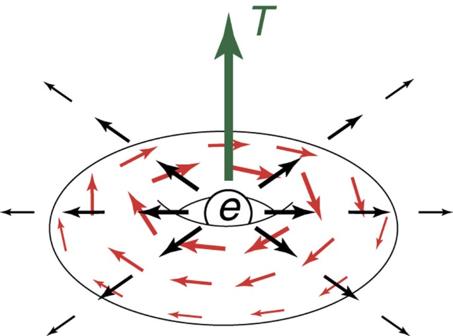Figure 3: Local toroic created around charge in magnetoelectric media. In magnetoelectrics with antisymmetric magnetoelectric tensor and with magnetic momentsM(r)~E(r) ×Tsuch object (‘magnetic donut’) will be created around electric chargee(close to the coreMshould decrease again). Thin radial arrows show the electric field, and red arrows show the orientation of magnetic moments around the chargee. Figure 3: Local toroic created around charge in magnetoelectric media. In magnetoelectrics with antisymmetric magnetoelectric tensor and with magnetic moments M ( r )~ E ( r ) × T such object (‘magnetic donut’) will be created around electric charge e (close to the core M should decrease again). Thin radial arrows show the electric field, and red arrows show the orientation of magnetic moments around the charge e . 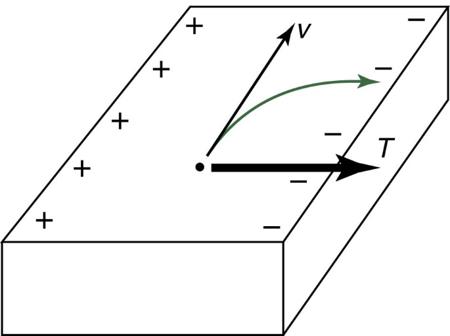Figure 4 Spontaneous Hall effect in media with toroidal momentT. Full size image Figure 4 Spontaneous Hall effect in media with toroidal moment T . Full size image Summarizing, I propose that nontrivial local magnetic objects, such as magnetic monopoles or magnetic toroics, should exist in magnetoelectric media in the bulk, associated with electrons or with charged impurities. Their presence can have unusual manifestations, such as an ‘electric Hall effect’ or a magnetophotovoltaic effect—effects that could be observable experimentally. Thus, the ME media can provide yet another possibility of modelling of magnetic monopoles in solids, more general and more easily detectable than, for example, in frustrated magnets [1] , [3] , [4] , [5] . One may expect many interesting effects in such systems, some of which were proposed above. Most of these can be explained both in the picture of magnetic monopoles and by the more traditional concepts, but the monopole picture is very transparent and illuminating, and it provides a natural language for discussing and predicting some novel nontrivial effects in magnetoelectric materials. It demonstrates that the electrodynamic response of these materials is even more interesting than usually assumed. It would also be interesting to compare the physics of monopoles in spin ice with that in magnetoelectrics and multiferroics. Very recently, the monopole characteristics in magnetoelectric systems were also discussed from a different perspective in ref. 17 , with the use of ab initio calculations for specific materials. I am grateful to N. A. Spaldin for informing me of this work. How to cite this article : Khomskii, D. I. Magnetic monopoles and unusual dynamics of magnetoelectrics. Nat. Commun . 5:4793 doi: 10.1038/ncomms5793 (2014).